A natural light-driven inward proton pump Light-driven outward H + pumps are widely distributed in nature, converting sunlight energy into proton motive force. Here we report the characterization of an oppositely directed H + pump with a similar architecture to outward pumps. A deep-ocean marine bacterium, Parvularcula oceani , contains three rhodopsins, one of which functions as a light-driven inward H + pump when expressed in Escherichia coli and mouse neural cells. Detailed mechanistic analyses of the purified proteins reveal that small differences in the interactions established at the active centre determine the direction of primary H + transfer. Outward H + pumps establish strong electrostatic interactions between the primary H + donor and the extracellular acceptor. In the inward H + pump these electrostatic interactions are weaker, inducing a more relaxed chromophore structure that leads to the long-distance transfer of H + to the cytoplasmic side. These results demonstrate an elaborate molecular design to control the direction of H + transfers in proteins. Microorganisms utilize ion-transporting rhodopsins such as light-driven pumps and light-gated channels for electrochemical membrane potential generation and signal transduction, respectively [1] . These rhodopsins are also important tools for optogenetics, which control neural activity by light [2] . While light-driven outward H + and inward Cl − pumps were discovered in the last century [3] , [4] , [5] , more recent metagenomic analyses led to the discovery of an outward Na + pump [6] , and cation [7] , [8] and anion channels [9] . 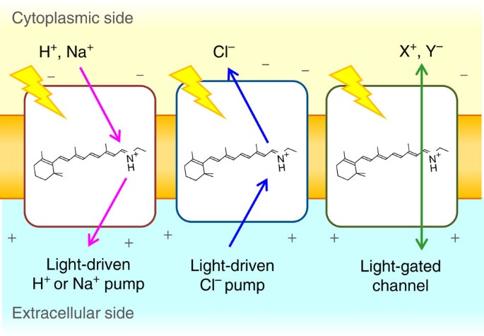Figure 1: Ion-transporting microbial rhodopsins. Light-driven outward cation pumps (left) and inward anion pumps (middle) function as active transporters, while light-gated channels conduct cations or anions in a passive manner (right). Figure 1 summarizes the functions of ion-transporting rhodopsins in which transport is uni-directional for pumps and bi-directional for channels [1] . The direction of transport for known retinal-binding ion pumps is exclusively outward for cations and inward for anions, increasing membrane potential. The presence of inward cation and outward anion pumps is highly unlikely in nature, as it is energetically unfavourable. Figure 1: Ion-transporting microbial rhodopsins. Light-driven outward cation pumps (left) and inward anion pumps (middle) function as active transporters, while light-gated channels conduct cations or anions in a passive manner (right). Full size image Previously, we engineered inward H + transport by mutating Anabaena sensory rhodopsin (ASR) [10] , a photochromic light sensor. Wild-type ASR does not transport ions, but an ASR mutant (D217E) exhibited light-induced inward H + transport when expressed in Escherichia coli cells. D217 is located in the cytoplasmic region of ASR, and light-induced difference Fourier transform infrared (FTIR) spectroscopy clearly showed an increased proton affinity for E217, which presumably controls the unusual directionality opposite to that in normal proton pumps. However, in that paper, we could not determine if the mutant functioned as an H + pump or channel as the inside of the cell was negatively charged. On a related note, conversions of light-driven outward H + pumps into an H + channel by mutation were reported recently [11] , [12] . Here we report that a microbial rhodopsin from a deep-ocean marine bacterium, Parvularcula oceani , functions as inward H + pump when expressed in E. coli and mouse neural cells. Mechanistic analyses of purified proteins reveal that the retinal chromophore structure and primary photoisomerization (C 13 =C 14 trans to cis ) are identical between outward and inward H + pumps. Nevertheless, the direction of primary H + transfer differs because of different electrostatic interactions of the protonated Schiff base with its counterion. We discuss these findings in terms of the molecular mechanisms of light-driven inward and outward H + pumps. Po XeR is a light-driven inward H + pump P. oceani is an α-proteobacterium found at a depth of 800 m in the south-eastern Pacific ocean. Analysis of the genome of P. oceani showed the existence of three microbial rhodopsins [13] . Two rhodopsins contain the NDQ and NTQ motifs, suggesting light-driven outward Na + ( Po NaR) and inward Cl − ( Po ClR) transport, respectively ( Fig. 2 ). The remaining rhodopsin possesses the DTL motif ( Fig. 2a ) and has amino-acid sequence 51% identical to that of ASR [14] , a photochromic light sensor ( Supplementary Fig. 1 ). Nevertheless, unlike ASR, this rhodopsin does not contain a long Arg-rich C-terminus ( Supplementary Fig. 1 ), and can be classified as a xenorhodopsin (XeR), whose function is unknown [15] ( Supplementary Fig. 1 ). Thus, unlike many microbes that normally contain an H + pump, P. oceani does not seem to have one. Instead, it has an Na + pump ( Po NaR), a Cl − pump ( Po ClR) and rhodopsin of an unidentified function ( Po XeR). 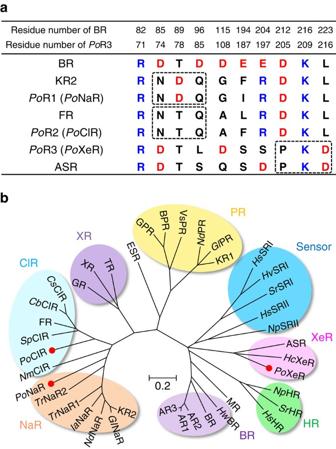Figure 2: Amino-acid sequence alignment of important residues and phylogenetic tree of microbial rhodopsins. (a) Important residues for the function of microbial rhodopsins. BR, KR2, FR and ASR are outward H+pump, outward Na+pump, inward Cl−pump, and photochromic sensor, respectively. Dashed rectangles indicate the positions of NDQ and NTQ motifs and residues unique for XeR. (b) Phylogenetic tree of selected microbial rhodopsins. The rhodopsins included in the phylogenetic tree: bacteriorhodopsin fromHalobacterium salinarum(BR), archaerhodopsin-1, -2 and -3 fromHalorubrum sodomense(AR1, AR2 and AR3), bacteriorhodopsin and middle rhodopsin fromHaloquadratum walsbyi(HwBR, MR), halorhodopsin fromH. salinarum,Salinibacter ruberandNatronomonas pharaonis (HsHR,SrHR,NpHR),PoXeR, xenorhodopsin fromHaloplasma contractile(HcXeR), ASR, sensory rhodopsin II fromN. pharaonisandH. salinarum(NpSRII andHsSRII), sensory rhodopsin I fromS. ruber,Haloarcula vallismortisandH. salinarum(SrSRI,HvSRI andHsSRI), proteorhodopsin fromKrokinobacter eikastus,Gillisia limnaea,Nonlabens dokdonensisandVibrio sp. AND4(KR1,GlPR,NdPR,VsPR), blue-absorbing proteorhodopsin from uncultured bacterium (BPR), green-absorbing proteorhodopsin from uncultured marine gamma proteobacterium (GPR), rhodopsin fromExiguobacterium sibiricum(ESR), thermophilic rhodopsin fromThermus thermophilus(TR), xanthorhodopsin fromS. ruber(XR), rhodopsin fromGloeobacter violaceus PCC 7421(GR), putative Cl−pumping rhodopsin fromCitromicrobium sp. JLT1363,Citromicrobium bathyomarinumandSphingopyxis baekryungensis(CsClR,CbClR,SpClR), Cl-pump fromFulvimarina pelagiandNonlabens marinus S1-08(FR andNmClR),PoClR,PoNaR, two putative NaRs fromTruepera radiovictrix(TrNaR1 andTrNaR2), putative NaR fromIndibacter alkaliphilus(IaNaR), NaR fromN. dokdonensis,G. limnaeaandK. eikastus(NdNaR,GlNaR and KR2). Figure 2: Amino-acid sequence alignment of important residues and phylogenetic tree of microbial rhodopsins. ( a ) Important residues for the function of microbial rhodopsins. BR, KR2, FR and ASR are outward H + pump, outward Na + pump, inward Cl − pump, and photochromic sensor, respectively. Dashed rectangles indicate the positions of NDQ and NTQ motifs and residues unique for XeR. ( b ) Phylogenetic tree of selected microbial rhodopsins. The rhodopsins included in the phylogenetic tree: bacteriorhodopsin from Halobacterium salinarum (BR), archaerhodopsin-1, -2 and -3 from Halorubrum sodomense (AR1, AR2 and AR3), bacteriorhodopsin and middle rhodopsin from Haloquadratum walsbyi ( Hw BR, MR), halorhodopsin from H. salinarum , Salinibacter ruber and Natronomonas pharaoni s ( Hs HR, Sr HR, Np HR), Po XeR, xenorhodopsin from Haloplasma contractile ( Hc XeR), ASR, sensory rhodopsin II from N. pharaonis and H. salinarum ( Np SRII and Hs SRII), sensory rhodopsin I from S. ruber , Haloarcula vallismortis and H. salinarum ( Sr SRI, Hv SRI and Hs SRI), proteorhodopsin from Krokinobacter eikastus , Gillisia limnaea , Nonlabens dokdonensis and Vibrio sp. AND4 (KR1, Gl PR, Nd PR, Vs PR), blue-absorbing proteorhodopsin from uncultured bacterium (BPR), green-absorbing proteorhodopsin from uncultured marine gamma proteobacterium (GPR), rhodopsin from Exiguobacterium sibiricum (ESR), thermophilic rhodopsin from Thermus thermophilus (TR), xanthorhodopsin from S. ruber (XR), rhodopsin from Gloeobacter violaceus PCC 7421 (GR), putative Cl − pumping rhodopsin from Citromicrobium sp. JLT1363 , Citromicrobium bathyomarinum and Sphingopyxis baekryungensis ( Cs ClR, Cb ClR, Sp ClR), Cl - pump from Fulvimarina pelagi and Nonlabens marinus S1-08 (FR and Nm ClR), Po ClR, Po NaR, two putative NaRs from Truepera radiovictrix ( Tr NaR1 and Tr NaR2), putative NaR from Indibacter alkaliphilus ( Ia NaR), NaR from N. dokdonensis , G. limnaea and K. eikastus ( Nd NaR, Gl NaR and KR2). Full size image We tested the ion-transporting functions of these rhodopsins using heterologous expression of C-terminally his-tagged proteins in E. coli . The membranes of Po NaR-expressing bacteria were yellow ( Fig. 3a ), suggesting low expression or improper folding of the protein. In contrast, Po ClR and Po XeR formed red/purple pigment ( Fig. 3a ). Next, we examined their ion-pumping activities. For Po ClR-expressing cells, we observed a light-induced increase in pH, which was accelerated by carbonylcyanide-m-chlorophenylhydrazone (CCCP) ( Fig. 3a ). This pH increase was similar in NaCl and CsCl, but was abolished when Na 2 SO 4 was used. Strong anion dependence is fully consistent with the inward Cl − pump function of Po ClR. For Po XeR-expressing cells, we also observed a light-induced pH increase in all salts, but the signals disappeared in the presence of CCCP ( Fig. 3a ). This suggests inward H + transport driven by light for Po XeR. Even though ASR does not transport ions [14] , we engineered inward H + transport of an ASR mutant (D217E) by light [10] . However, it was not clear D217E ASR is an inward H + pump or channel, because the inside of the cell is negatively charged. To verify the active nature of inward proton transport, voltage and current across the membrane should be controlled. For this purpose, we expressed Po XeR in mouse ND7/23 cells and performed electrophysiological measurements. The data in Fig. 3b display an inward current for all measured membrane voltages (from −55 mV to 45 mV). More importantly, the obtained I – V curve was identical for different extracellular pH values (7.2 and 9.0), typical for light-driven H + pumps. Thus, despite the lack of measurements in native cells, the results in E. coli and ND7/23 cells strongly suggest that Po XeR is a natural light-driven inward H + pump. 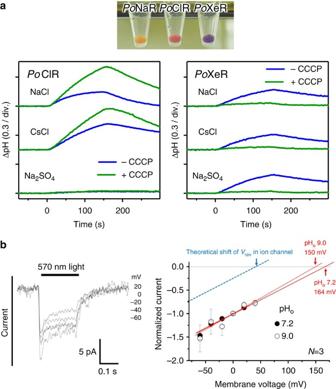Figure 3: Light-driven H+transport activity ofPoXeR. (a)E. coliC43(DE3) strain cells in which the expression ofPoNaR,PoClR andPoXeR was induced (upper), and ion-pumping activity was assayed by observing pH changes (lower). Light is on between 0 and 150 s. (b) Electrophysiological measurements ofPoXeR-driven photocurrent in ND7/23 cells (left) andI–Vplot of the current at pHo7.2 and 9.0. Figure 3: Light-driven H + transport activity of Po XeR. ( a ) E. coli C43(DE3) strain cells in which the expression of Po NaR, Po ClR and Po XeR was induced (upper), and ion-pumping activity was assayed by observing pH changes (lower). Light is on between 0 and 150 s. ( b ) Electrophysiological measurements of Po XeR-driven photocurrent in ND7/23 cells (left) and I – V plot of the current at pH o 7.2 and 9.0. Full size image Molecular properties of Po XeR The unusual inward H + pumping activity of Po XeR poses questions about its physiological role and molecular mechanism. The former is difficult to address as the culture of native cells is not available. As for the latter, we studied the molecular mechanism of the inward H + pumping by various spectroscopic methods using Po XeR expressed in E. coli . 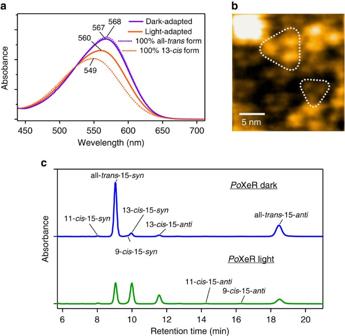Figure 4: Molecular properties ofPoXeR. (a) Absorption spectra of dark- and light-adaptedPoXeR (purple and orange solid lines, respectively). Dashed lines represent the calculated spectra of 100% all-transand 100% 13-cisforms. (b) High-speed AFM image ofPoXeR reconstituted in a nanodisc. (c) HPLC pattern of retinal extracted fromPoXeR. Figure 4a shows the absorption spectrum of Po XeR ( λ max =567 nm) in the dark and after illumination, and a high-speed atomic force microscopy (AFM) image ( Fig. 4b ) shows that Po XeR forms a trimer in the nanodisk membrane. ASR contains predominantly all- trans chromophore in the dark but the 13- cis , 15- syn chromophore is formed after light-adaptation [16] , [17] . This is also the case for Po XeR, which is 92% all- trans in the dark while all- trans and 13- cis forms are equally distributed after the illumination ( Fig. 4c ). Calculated absorption spectra of all- trans and 13- cis forms exhibit λ max at 568 and 549 nm, respectively, similar to those observed for ASR [18] . Figure 4: Molecular properties of Po XeR. ( a ) Absorption spectra of dark- and light-adapted Po XeR (purple and orange solid lines, respectively). Dashed lines represent the calculated spectra of 100% all- trans and 100% 13- cis forms. ( b ) High-speed AFM image of Po XeR reconstituted in a nanodisc. ( c ) HPLC pattern of retinal extracted from Po XeR. Full size image Photoreaction dynamics of a dark-adapted Po XeR We next studied the photocycle of the dark-adapted Po XeR protein, which presumably represents the inward H + pumping process. To avoid photoexcitation of the 13- cis form, we measured single-wavelength kinetics of a 0.6 ml sample of dark-adapted protein, and replaced it after each single excitation measurement. 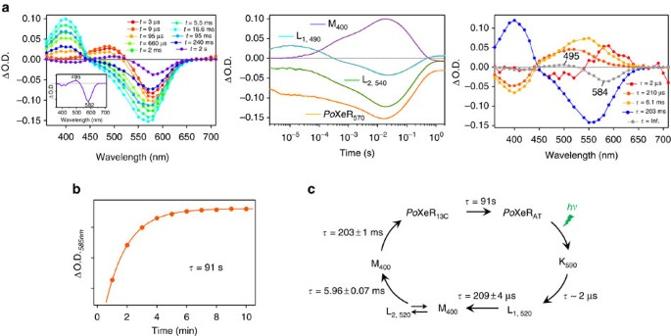Figure 5: Photoreaction dynamics ofPoXeR. (a) Transient difference absorption spectra of dark-adaptedPoXeR (left) and absorption difference time-evolution at specific wavelengths (centre). Decay-associated spectra obtained by global fitting of the changes in transient absorption (right). The inset shows the difference spectrum between light-adapted and dark-adapted state. (b) The process of dark-adaptation estimated by the recovery of absorption at 585 nm. (c) The photocycle ofPoXeR. Values of the time-constants of each process are the mean±s.d. Figure 5a shows the time-resolved difference spectra (left), absorption changes at each wavelength (centre) and decay-associated spectra (right). Upon photoexcitation of the all- trans form ( Po XeR AT ), the red-shifted K intermediate appears first, and decays to the blue-shifted L intermediate in 2 μs. Then, the M intermediate containing a deprotonated Schiff base appears with two distinct time-constants (210 μs and 6.0 ms). This analysis shows the presence of two states for L and M, one of which is in equilibrium. The M-intermediate decays in 200 ms, but the transient absorption does not return to zero ( Fig. 5a , centre) at >1 s, indicating the presence of another long-lived intermediate state. The difference spectrum obtained by transient absorption spectroscopy (spectrum at 2 s in Fig. 5a , left) coincides with that obtained by steady-state absorption measurements in Fig. 4a ( Fig. 5a , inset). Therefore, the last intermediate represents metastable 13- cis state ( Po XeR 13C ) that reverts into Po XeR AT in 91 s ( Fig. 5b ). The photocycle of Po XeR AT is summarized in Fig. 5c : the inward H + transport is made possible by (i) H + release from the Schiff base to the cytoplasmic region upon M formation and (ii) H + uptake from the extracellular region upon M decay. Figure 5: Photoreaction dynamics of Po XeR. ( a ) Transient difference absorption spectra of dark-adapted Po XeR (left) and absorption difference time-evolution at specific wavelengths (centre). Decay-associated spectra obtained by global fitting of the changes in transient absorption (right). The inset shows the difference spectrum between light-adapted and dark-adapted state. ( b ) The process of dark-adaptation estimated by the recovery of absorption at 585 nm. ( c ) The photocycle of Po XeR. Values of the time-constants of each process are the mean±s.d. Full size image H + pathway during the inward transport in Po XeR As light-driven outward H + pumps contain internal H + acceptors and donors [1] , we examined candidates for such groups for the inward H + pump. Membrane-embedded carboxylates are strong candidates for internal H + acceptors and donors, as is the case for D85 (acceptor) and D96 (donor) in an outward H + pump BR (refs 19 , 20 ). 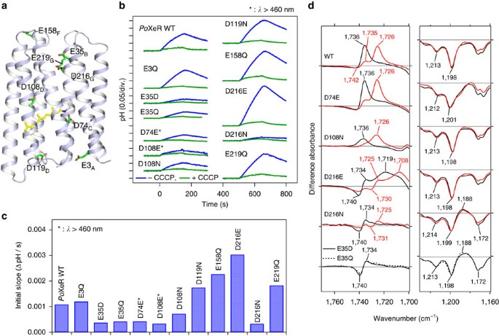Figure 6: Inward H+pumping activity and light-induced FTIR spectra ofPoXeR and its mutants. (a) The crystal structure of ASR (PDB ID: 1XIO)21is shown with the side chains of the acidic residues used inPoXeR mutagenesis studies. The residue numbering of PoXeR is shown. (b) H+transport activity ofPoXeR mutants inE. colicells after normalization for the amount of protein. Light is on between 0 and 150 s. (c) The initial slopes of light-induced pH changes shown inb. (d) Light-induced difference FTIR spectra of WTPoXeR and the mutants atT=230 K and pH 8.0. Spectra are measured in H2O (black) and D2O (red). Figure 6a shows putative location of eight intramembrane carboxylates possibly involved in the transport, which we replaced with neutral residues (D-to-N or E-to-Q). Among the mutants, only D74N showed the absence of colour. As D74 acts as the counterion of the protonated Schiff base, we attempted a more conservative replacement, D74E. The inward H + pumping activity was measured for various mutants ( Fig. 6b ), and the initial slopes are plotted in Fig. 6c . Figure 6: Inward H + pumping activity and light-induced FTIR spectra of Po XeR and its mutants. ( a ) The crystal structure of ASR (PDB ID: 1XIO) [21] is shown with the side chains of the acidic residues used in Po XeR mutagenesis studies. The residue numbering of PoXeR is shown. ( b ) H + transport activity of Po XeR mutants in E. coli cells after normalization for the amount of protein. Light is on between 0 and 150 s. ( c ) The initial slopes of light-induced pH changes shown in b . ( d ) Light-induced difference FTIR spectra of WT Po XeR and the mutants at T =230 K and pH 8.0. Spectra are measured in H 2 O (black) and D 2 O (red). Full size image The results clearly show a significant reduction in the pumping activity in E35D/Q, D74E, D108E/N and D216N. In contrast, D216E showed about threefold higher inward H + pumping activity than wildtype (WT). It should be noted that the corresponding mutant of ASR (D217E) shows inward H + transport [10] . Previously, light-induced difference FTIR spectroscopy of D217E ASR revealed protonation of E217 upon deprotonation of the Schiff base (M intermediate) [10] . Here we applied similar FTIR analysis to Po XeR AT ( Supplementary Fig. 2 ). The top panel of Fig. 6d shows a positive peak at 1,736 cm −1 , which down-shifts to 1,726 cm −1 in D 2 O in the M-minus- Po XeR AT difference spectra. This is a characteristic signal of protonated carboxylic acids, indicating that carboxylate is the H + acceptor of the Schiff base. Similar positive peaks were observed for D74E and D108N, but an entirely different spectral feature was obtained for D216E. Sharp positive peaks of WT at 1,736 and 1,726 cm −1 in H 2 O and D 2 O were shifted to 1,719 and 1,708 cm −1 in D216E, respectively, and the remaining pair of peaks at 1740 (−)/1734 (+) cm −1 in H 2 O (1,730 (−)/1,725 (+) cm −1 in D 2 O) originates from a different carboxylic acid. This strongly suggests that D216 is the H + acceptor during the inward H + transport in Po XeR. In agreement with that idea, the positive peak at 1,736 cm −1 was absent in D216N. In contrast, a positive peak was observed at 1,188 cm −1 in the C–C stretching region of retinal chromophore, indicating that the M intermediate did not form in D216N. There was no positive peak in the frequency region of protonated carboxylic acids and the 1,188 cm −1 band was present (no M formation) in E35Q/D as well. From homology modelling, E35 is likely to be located near D216, and the E35 mutation may raise the pKa of D216, leading to the lack of M formation. According to the structure of ASR, the distance between the Schiff base and D217 (D216 in Po XeR) is 14.7 Å (ref. 21 ), and such long-range H + transfer should be mediated by other residues and/or water molecules in the inward H + pump. As for the identity of H + donor to the Schiff base, the decay of the M intermediate accompanies protonation of the Schiff base, and if H + is taken up from the aqueous phase, the decay of M should slow down at high pH (ref. 22 ). We thus measured the M decay kinetics at different pH values. 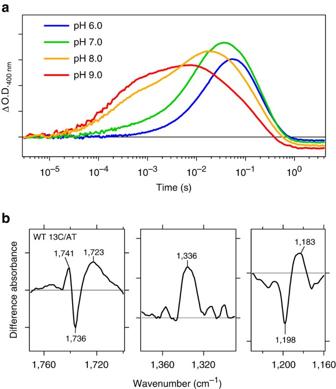Figure 7: Analysis of H+uptake inPoXeR. (a) Time-evolution of the accumulation of M intermediate at various pH values. (b) Light-induced difference FTIR spectra betweenPoXeR13CandPoXeRATstates at 277 K and pH 8.0. Figure 7a shows strong pH dependence of the M rise but limited pH dependence of the M decay. In fact, the speed of M decay increased at pH 9.0. This fact indicates the presence of an internal H + donor. If it is a carboxylic acid, we expect a negative band in the 1,760–1,700 cm −1 region in the Po XeR 13C -minus- Po XeR AT difference FTIR spectra. However, Fig. 7b shows a broad positive peak at 1,723 cm −1 in addition to a peak pair at 1,741 (+)/1,736 (−) cm −1 . Absence of deprotonation signal in this region questions the role of a carboxylic acid as the H + donor. Other residues such as arginine and protein-bound water molecules are possible candidates for the internal H + donor [23] , [24] . The spectral features at 1,336 (+) cm −1 and 1,198 (−)/1,183 (+) cm −1 ( Fig. 7b and Supplementary Fig. 3 ) resemble those of the dark adaptation in BR [25] , suggesting that Po XeR 13C contains the 13- cis , 15- syn configuration. Figure 7: Analysis of H + uptake in Po XeR. ( a ) Time-evolution of the accumulation of M intermediate at various pH values. ( b ) Light-induced difference FTIR spectra between Po XeR 13C and Po XeR AT states at 277 K and pH 8.0. Full size image In this paper, we report the discovery and characterization of a natural retinal-binding inward H + pump ( Po XeR). Mechanistic analyses of the purified protein revealed that the retinal chromophore structure and primary photoisomerization (C 13 =C 14 trans to cis ) are identical between outward and inward H + pumps. Nevertheless, direction of the primary H + transfer in Po XeR is opposite to that in outward H + pumps. The pathway of the inward H + transport in Po XeR is summarized in Fig. 8 . The primary H + transfer occurs from the Schiff base to D216 on the cytoplasmic side. E35 modulates its pKa by forming hydrogen-bonding network with D216, similar to the one reported for ASR (E36 and D217) [26] . Secondary H + transfer occurs from an unidentified group to the Schiff base on the extracellular side. This sequence of events in H + transport is entirely opposite to the one well-known for outward H + pumps such as BR [1] , [27] , [28] , [29] , [30] , [31] , [32] , [33] . 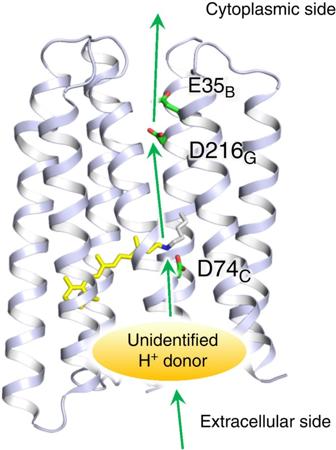Figure 8: Model for H+transfer pathway inPoXeR. The H+transfer pathway inPoXeR suggested by the results of the present study. The primary H+transfer occurs from the Schiff base to D216, and E35 affects this reaction. The Schiff base is not directly reprotonated from the aqueous phase, but there is an internal H+donor, yet to be identified. Figure 8: Model for H + transfer pathway in Po XeR. The H + transfer pathway in Po XeR suggested by the results of the present study. The primary H + transfer occurs from the Schiff base to D216, and E35 affects this reaction. The Schiff base is not directly reprotonated from the aqueous phase, but there is an internal H + donor, yet to be identified. Full size image We suggest the following mechanism for the distinct vectoriality between Po XeR and BR transport ( Fig. 9 ). Photoexcitation first converts the all- trans chromophore into a twisted 13- cis , 15- anti state in both, but its relaxation differs between BR and Po XeR. There are two negative charges, D85 and D212, on the extracellular side of BR, producing strong electrostatic attraction of the protonated Schiff base before the primary H + transfer, leading to outward H + transport [34] . In contrast, the XeR family possesses only one negative charge in that region, as D212 of BR is replaced by proline, which makes the electrostatic interaction between the protonated Schiff base and the counterion (D74 in Po XeR) weaker [35] , [36] , [37] , [38] . Consequently, photoisomerization reorients the N–H group of the Schiff base toward the cytoplasmic side. The cytoplasmic domain is more polar in ASR than in BR [21] , and such a structure should promote long-distance H + transfer to D216 in Po XeR. 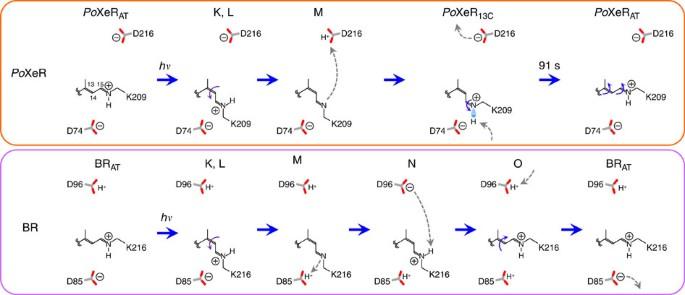Figure 9: Mechanism of inward H+transport inPoXeR and outward H+transport in BR. Schematic description of H+transport in the photocycle ofPoXeR compared with the photocycle of BR. In BR, only one double bond at C13=C14isomerizes during the outward H+pumping photocycle (transtocisphotoisomerization, andcistotransthermal isomerization). In contrast, retinal isomerization is more complex to facilitate the inward H+pump inPoXeR: (i) C13=C14transtocisphotoisomerization, (ii) C15=Nantitosynthermal isomerization, and (iii) C13=C14cistotransand C15=Nsyntoantithermal isomerization by a bicycle-pedal motion. Figure 9: Mechanism of inward H + transport in Po XeR and outward H + transport in BR. Schematic description of H + transport in the photocycle of Po XeR compared with the photocycle of BR. In BR, only one double bond at C 13 =C 14 isomerizes during the outward H + pumping photocycle ( trans to cis photoisomerization, and cis to trans thermal isomerization). In contrast, retinal isomerization is more complex to facilitate the inward H + pump in Po XeR: (i) C 13 =C 14 trans to cis photoisomerization, (ii) C 15 =N anti to syn thermal isomerization, and (iii) C 13 =C 14 cis to trans and C 15 =N syn to anti thermal isomerization by a bicycle-pedal motion. Full size image After the M-intermediate formation, BR receives H + from the cytoplasmic side, followed by thermal isomerization to the original all- trans form. Therefore, only one double bond at C 13 =C 14 bond isomerizes during the functional photocycle of BR. In contrast, after M formation of Po XeR, it is likely that thermal isomerization occurs at C 15 =N bond from an anti to a syn form, followed by secondary H + transfer on the extracellular side. This yields a 13- cis , 15- syn form ( Po XeR 13C ), and thermal bicycle-pedal isomerization [39] (13- cis , 15- syn to all- trans , 15- anti ) reverts it to the original state. Thermal isomerization of the C 15 =N group was known for BR as a dark-adaptation process [25] , but is directly related to the function of XeRs, such as ASR and Po XeR. In ASR, C 15 =N thermal isomerization after C 13 =C 14 photoisomerization occurs with 100% yield, leading to an efficient photochromic reaction [18] , [40] . In Po XeR, C 15 =N thermal isomerization allows for an inward H + transport, an additional function for microbial rhodopsins, though the thermal isomerization yield is unknown at present. Inward H + transport may lower the proton motive force, which is bioenergetically disadvantageous for marine bacteria. Thus, its presence in nature suggests a different physiological role, not related to bioenergetics. One possibility is that the inward H + pump may be used for intracellular signal transduction, similar to ASR [14] . A future structure–function study of Po XeR should lead to a better understanding of this unique function. The light-driven inward H + pump is also a potential tool for optogenetics. The light-driven outward H + pump Arch has been used as a neural silencer in optogenetics and Arch is also used for acidification of cell organelles [41] . An oppositely directed light-driven H + pump would further enable the control of cell organelles. In summary, we show that Po XeR is a light-driven inward H + pump from a marine α-proteobacterium. While outward H + pumps are widely present in nature, oppositely directed H + pumps are rare. In inward H + pumps, the lack of a negative charge in the active centre causes weak coupling to the Schiff base counterion (D74) in the key photocycle intermediate, leading to the release of H + to D216 in the cytoplasmic region. Retinal isomerization sequence became more complex to facilitate the inward H + transport: (i) C 13 =C 14 trans to cis photoisomerization, (ii) C 15 =N anti to syn thermal isomerization and (iii) C 13 =C 14 cis to trans and C 15 =N syn to anti thermal isomerization by a bicycle-pedal motion [39] . This work demonstrates an elaborate molecular design to control the direction of H + transport in retinal-binding proteins. The discovery of a light-driven inward H + pump will lead to better understanding of the molecular mechanism of light-driven pumps and contribute to the development of new optogenetic tools. Protein expression and purification Genes of Po XeR, Po NaR and Po ClR, whose codons were optimized for an E. coli expression system, were synthesized (Eurofins Genomics Inc.) and subcloned into a pET21a(+)-vector with C-terminal 6 × His-tag. For mutagenesis, a QuikChange site directed mutagenesis kit (Stratagene) was used according to a standard protocol. Wildtype and mutant proteins were expressed in E. coli C43(DE3) strain. Protein expression was induced by 0.21 mM isopropyl β- D -thiogalactopyranoside (IPTG) for 4 h at 37 °C when 10 μM all- trans -retinal (Sigma-Aldrich) was supplemented in the culture. The expressed proteins were purified from E. coli cells using previously reported protocols [6] , [42] , [43] , [44] . The cells were disrupted by a French Press (Ohtake) and the membrane fraction was collected by ultracentrifugation (125,000 g , 1 h). The protein was solubilized with 2% n -dodecyl-β- D -maltoside (DDM) (Anatrace) in the presence of 300 mM NaCl, 5 mM imidazole and 50 mM MES (pH 6.5). After Co 2+ -NTA affinity chromatography, the collected fractions were dialyzed against a solution containing 50 mM Tris–HCl pH 8.0, 100 mM NaCl, 0.1% DDM to remove imidazole used for the elution from a column. Assay of light-driven ion-pumping activity of rhodopsins E. coli cells expressing rhodopsins were collected by centrifugation (4,800 g , 3 min), washed three times with and resuspended in aqueous solution containing 100 mM salt (NaCl, CsCl and Na 2 SO 4 ). Cell suspension of 7.5 ml at OD 660 =2 was placed in the dark and then illuminated at λ >500 nm by a 1-kW tungsten–halogen projector lamp (Rikagaku, Japan) through a glass filter (Y-52, AGC Techno Glass, Japan). For the blue-shifted Po XeR mutants ( Po XeR D74E and D108E), light of λ >460 nm (Y-48, AGC Techno Glass, Japan) was used for the photoexcitation. The light-induced pH changes were measured by a pH electrode (HORIBA, Japan). Measurements were repeated under the same conditions after the addition of 10 μM CCCP. Quantification of rhodopsins expressed in E. coli The amount of rhodopsin expressed in E. coli was estimated by a previously reported method [6] , [43] , [44] . E. coli cells expressing rhodopsins were collected by centrifugation at 3,600 g and 4 °C and suspended in a solution containing 100 mM NaCl and 50 mM Tris–HCl (pH 8.0), to a final volume of 3 ml. Then, 200 μl of 1 mM lysozyme was added to the suspension and it was gently stirred at room temperature for 1 h. The E. coli cells were disrupted by sonication (TAITEC, Japan) and solubilized in 3.0% DDM. The change in absorption, which represents the bleaching of rhodopsin by hydroxylamine (HA), was measured with a ultraviolet–vis spectrometer (Shimadzu, Japan) equipped with an integrating sphere after the addition of HA to a final concentration of 500 mM and illumination at λ >500 nm by a 1-kW tungsten–halogen projector lamp (Rikagaku, Japan) through a glass filter (Y-52, AGC Techno Glass, Japan). The molecular extinction coefficient of WT Po XeR and mutant proteins ( ɛ ) was calculated from the ratio between the absorbance of rhodopsin and retinal oxime ( ɛ =33,600 M −1 cm −1 at 360 nm (ref. 45 ) produced by the reaction between the retinal Schiff base and HA. The amount of protein expressed in E. coli cells was determined by the absorbance of the bleached rhodopsin. The transport activity of E. coli cells containing each rhodopsin was quantitatively determined from the initial slope of pH change after normalizing by the expression level of protein. Measurement of dark-adaptation kinetics Dark adaptation kinetics was measured for 0.1% DDM-solubilized sample at 24 °C. The dark-adapted sample was illuminated for 2 min by using output from a 1-kW tungsten–halogen projector lamp (Master HILUX-HR, Rikagaku, Japan) through a glass filter (O-60, AGC Techno Glass, Japan) at λ >580 nm. After turning off the light, the spectra or the absorption at a specific wavelength were measured every 1 min or 1 s, respectively, by a ultraviolet–visible spectrometer (V-730, JASCO). Heterologous expression in mammalian cells A human codon-adapted Po XeR gene was synthesized by Gen Script (Piscataway, NJ, USA) and cloned into pEGFP vector between Hind III and Bam HI sites. ND7/23 cells were purchased from DS Pharma Biomedical (Osaka, Japan) and cultured in high-glucose DMEM media (Wako) in a 37 °C, 5% CO 2 incubator. Transfection of ND7/23 cells was performed by Lipofectamine 2000 (Invitrogen, Carlsbad, CA, USA). Cells were supplemented with 1 μM all- trans -retinal (Sigma-Aldrich) after transfection. Expression was confirmed by a fluorescence microscope (IX-73, Olympus, Tokyo, Japan). Electrophysiology Whole cell patch clamp was performed with an amplifier, Axopatch 200B (Molecular Devices, Sunnyvale, CA, USA). Continuous light was provided by OSG L12194-00-39070 (Hamamatsu Photonics, Shizuoka, Japan) via a light guide into an inverted microscope, IMT-2 (Olympus, Tokyo Japan). Illumination was controlled by a mechanical shutter LS6S (Vincent Associates, Rochester, NY, USA). Glass pipettes were fabricated by a micropipette puller, P-97 (Sutter Instrument, Novato, CA, USA) and fire-polished by a micro forge, MF-830 (Narishige, Tokyo, Japan). The pipette resistance was 1.5–2.5 MΩ. The pipette electrode was controlled by a micro manipulator, PCS-5000 (Burleigh instruments, Fishers, NY, USA). Current traces were recorded at 10 kHz and filtered to 2 kHz by an internal circuit of the amplifier. Data acquisition and shutter triggering were performed by pClamp 10 software via a Digidata 1550 (Molecular Devices, Sunnyvale, CA, USA). Data were analysed by Clampfit 10 software. The standard external solution contained 140 mM NaCl, 2 mM MgCl 2 , 2 mM CaCl 2 , 2 mM KCl and 10 mM HEPES-NaOH (pH 7.2). The standard internal solution contained 110 mM NaCl, 2 mM MgCl 2 , 1 mM CaCl 2 , 5 mM KCl, 10 mM EGTA and 10 mM HEPES-NaOH (pH 7.2). Osmolality of the solutions was adjusted to 300 mOsm by adding an appropriate amount of sucrose. Preparation of Po XeR reconstituted in asolectin For Po XeR reconstitutions in a lipid bilayer, we used a nanodisc protocol [46] , [47] , [48] . Briefly, Po XeR ( ∼ 5 nM) solubilized in 0.1% DDM, membrane scaffold proteins (MSP1E3D1) (M7074, Sigma) ( ∼ 30 μM) and asolectin (11145, Sigma) ( ∼ 120 μg) were mixed in a solution containing 20 mM HEPES (pH 7.4) and 100 mM NaCl. The mixture was incubated for 1 h at 4 °C and then Bio-Beads SM-2 (Bio-Rad) (60 mg) were added to remove the detergent. After mixing overnight at 4 °C, Bio-Beads were removed by centrifugation at 14,000 r.p.m. and 4 °C for 1 min. The nanodisc products were purified by a 0.45 μm syringe filter (Millipore). High-speed AFM In-house high-speed AFM operated in tapping mode was used [49] , [50] . In high-speed AFM, the cantilever deflection is detected by an optical beam deflection detector using an infrared laser (780 nm). The laser beam is focused onto the back side of a cantilever covered by a gold film through a × 60 objective lens (Nikon: CFI S Plan Fluor ELWD 60 × ) and the reflected laser is detected by a two-segmented PIN photodiode. The size of a cantilever (Olympus: BL-AC7DS-KU4) is 6–7 μm long, 2 μm wide, and 90 nm thick. A spring constant is estimated to be 0.1–0.2 N m −1 by a thermal method, and a resonant frequency and quality factor of a cantilever in liquid are ∼ 1 MHz and ∼ 2, respectively. The free oscillation amplitude was ∼ 1 nm and the set-point amplitude was about 90% of the free amplitude during the AFM observation. To gain a sharp probe, we deposited an amorphous carbon tip on the initial bird’s beak tip by electron beam deposition. The length of an amorphous carbon tip was ∼ 500 nm, and the end radius of the tip was ∼ 4 nm. The AFM was performed under the buffer solution containing 20 mM Tris–HCl (pH 8.0) and 100 mM NaCl at room temperature. HPLC analysis of retinal configuration The configuration of retinal in Po XeR was analysed by high-performance liquid chromatograph (HPLC) as described previously [17] . A silica column (6.0 × 150 mm; YMC-Pack SIL) was used for the analysis. We added HA (final conc. 500 mM) to 100 μl Po XeR solution (100 mM NaCl, 20 mM Tris–HCl (pH 8.0)) at 4 °C, and then the protein was denatured with 66% (v/v) methanol. The retinal of Po XeR was released as retinal-oxime and extracted with hexane. The extracted sample was analysed by HPLC (solvent composition: 12% (v/v) ethyl acetate and 0.12% (v/v) ethanol in hexane) with 1.0 ml min −1 flow rate. The molar fraction of each retinal isomer was calculated from the ratio of the areas of corresponding peaks in the HPLC patterns. Each peak was assigned by comparison with the HPLC pattern of retinal oximes obtained from pure free all- trans - and 13- cis retinals. To analyse the retinal configuration of light-adapted Po XeR, the sample solution was illuminated with λ >500 nm light (Y-52, AGC Techno Glass) for 1 min before the reaction with HA at 4 °C. To estimate the experimental error, three identical measurements were performed for both dark- and light-adapted samples. Laser flash photolysis The time-evolution of the transient absorption changes of photo-excited Po XeR was observed as previously described [6] . The purified sample was resuspended in buffer containing 50 mM Tris–HCl (pH 8.0), 100 mM NaCl and 0.1% DDM. The sample solution was placed in a quartz cuvette and was excited with a beam of second harmonics of a nanosecond pulsed Nd 3+ :YAG laser ( λ =532 nm, INDI40, Spectra-Physics). The excitation laser power was 3 mJ pulse −1 . Sample solution of 0.6 ml was used for each measurement and was replaced by a fresh dark-adapted sample for every photoexcitation. The change in transient absorption after photoexcitation was obtained by observing the change of the intensity of monochromated output of a Xe arc lamp (L9289-01, Hamamatsu Photonics, Japan) passed through the sample by a photomultiplier tube (R10699, Hamamatsu Photonics, Japan). Transient absorption spectra were reconstructed from the time-evolution of the change in transient absorption at various wavelengths from 360 to 710 nm with 10-nm intervals. The signals were global-fitted with a multi-exponential function and decay-associated spectra were obtained by plotting the pre-exponential factors against probed wavelengths. Low-temperature difference FTIR spectroscopy For FTIR spectroscopy, WT Po XeR and mutants were reconstituted into a mixture of POPE and POPG (molar ratio=3:1) with a protein-to-lipid molar ratio of 1:50 by removing DDM with Bio-Beads (SM-2, Bio-Rad). The reconstituted samples were washed three times with 1 mM NaCl and 2 mM Tris–HCl (pH 8.0). The pellet was resuspended in the same buffer, but the concentration was adjusted to 1.7 mg ml −1 . A 60 μl aliquot was placed onto a BaF 2 window and dried with an aspirator. Low-temperature FTIR spectroscopy was applied to the films hydrated with H 2 O and D 2 O at 230 and 277 K as described previously [10] , [51] , [52] . For the formation of the M intermediate, samples were illuminated with >500 nm light for 1 s. To measure the difference infrared spectrum between Po XeR AT and Po XeR 13C , the latter was accumulated with >590-nm light for 1 min and spectra were measured during illumination. For each measurement, 128 interferograms were accumulated, and 2–4 identical recordings were averaged. Phylogenic analysis of rhodopsin genes The amino-acid sequences of rhodopsins were aligned using MUSCLE programme [53] after the removal of a weakly conserved interhelical loop, and N- and C-terminal extensions to increase the accuracy of alignment. The evolutionary history was inferred using the Neighbor-Joining method [54] . The optimal phylogenetic tree with the sum of branch length=15.12577349 was obtained. The percentage of replicate trees in which the associated taxa clustered together in the bootstrap test (1,000 replicates) were calculated [54] . The tree is drawn to scale, with branch lengths in the same units as those of the evolutionary distances used to infer the phylogenetic tree. The evolutionary distances were computed using the Poisson correction method [55] and the units are the number of amino-acid substitutions/site. The analysis involved 41 amino-acid sequences. All positions containing gaps and missing data were eliminated. There were a total of 126 positions in the final dataset. Evolutionary analyses were conducted in MEGA6 (ref. 56 ). Data availability The data that support the findings of this study are available from the corresponding author upon reasonable request. The structures of BR (PDB ID: 1M0L) and ASR (PDB ID: 1XIO) were used to highlight residues in transmembrane helices in Supplementary Fig. 1 and for illustrations purposes in Fig. 6 and Fig. 8 . How to cite this article: Inoue, K. et al . A natural light-driven inward proton pump. Nat. Commun. 7, 13415 doi: 10.1038/ncomms13415 (2016). Publisher's note: Springer Nature remains neutral with regard to jurisdictional claims in published maps and institutional affiliations.